Synthetic lateral inhibition governs cell-type bifurcation with robust ratios Cell-type diversity in multicellular organisms is created through a series of binary cell fate decisions. Lateral inhibition controlled by Delta–Notch signalling is the core mechanism for the choice of alternative cell types by homogeneous neighbouring cells. Here, we show that cells engineered with a Delta–Notch-dependent lateral inhibition circuit spontaneously bifurcate into Delta-positive and Notch-active cell populations. The synthetic lateral inhibition circuit comprises transcriptional repression of Delta and intracellular feedback of Lunatic fringe (Lfng). The Lfng-feedback subcircuit, even alone, causes the autonomous cell-type bifurcation. Furthermore, the ratio of two cell populations bifurcated by lateral inhibition is reproducible and robust against perturbation. The cell-type ratio is adjustable by the architecture of the lateral inhibition circuit as well as the degree of cell–cell attachment. Thus, the minimum lateral inhibition mechanism between adjacent cells not only serves as a binary cell-type switch of individual cells but also governs the cell-type ratio at the cell-population level. Diverse cell types in a multicellular organism arise from a single fertilized egg. This fact indicates that cell-type diversification occurs repeatedly throughout development. An important mechanism for creating a difference among initially homogeneous cells is lateral inhibition, a mutual inhibition mechanism between adjacent cells that is mediated by Delta–Notch signalling [1] , [2] , [3] , [4] . Both the ligand Delta and its receptor Notch are transmembrane proteins, and ligand–receptor binding between adjacent cells causes activation and subsequent cleavage of Notch. The released Notch intracellular domain (NICD) acts as a transcriptional regulator, leading to the downregulation of Delta expression. Thus, production of Delta in one cell represses the transcription of Delta in the adjacent cells. The mutual transcriptional repression of Delta between adjacent cells is called lateral inhibition, which is equivalent to an intercellular (double-negative) positive feedback loop. As such, a cell–cell positive feedback loop has the ability to amplify a small initial difference between cells [5] , [6] , [7] , [8] , initially homogeneous adjacent cells can become radically different, eventually settling down in a pair of stable steady states: a Delta-on/Notch-off state and Delta-off/Notch-on state. Then, the cells with distinct Delta–Notch states adopt different cell fates. A prominent example of the binary cell fate decision through lateral inhibition is the specification of bristle precursor cells in initially homogeneous epithelial cells in Drosophila [3] , [4] , [9] , [10] , [11] . In vertebrates, the lateral inhibition mechanism also governs cell fate decisions between neurons and non-neuronal cells in the central nervous system [3] , [12] , [13] , [14] , secretory cells and absorptive cells in the intestine [15] , [16] , [17] , [18] , and hair cells and supporting cells in the inner ear [3] , [19] , [20] . As these mechanisms and roles of lateral inhibition have been revealed mainly by disruption experiments, where the cell fate decision processes were disturbed by inhibition or overexpression of the components of Delta–Notch signaling, it has been difficult to identify sufficient conditions for lateral inhibition to create a stable difference between cells. For example, lateral inhibition by Delta–Notch signalling often accompanies asymmetric cell division (that is, unequal distribution of regulatory molecules between daughter cells) [21] , [22] . Whether lateral inhibition can create an enough difference without the help of asymmetric cell division has been unclear. In this study, inspired by the lateral inhibition mechanism in vivo , we aim to create a minimum genetic circuit that would cause spontaneous cell-type bifurcation between adjacent cells. We demonstrate that our synthetic lateral inhibition circuit, which comprises only four genetic components, not only gives rise to two distinct cell types but also maintains an appropriate ratio of the two cell types at the cell-population level without any external cues. Design and construction of lateral inhibition circuits All of the genetic circuits were constructed in Chinese hamster ovary (CHO) cells, which do not have a native lateral inhibition mechanism. CHO cells do not express endogenous Delta and express only a small amount of endogenous Notch [23] . We first constructed a basic transcriptional repression (bTR) circuit ( Fig. 1a ). When Delta binds to weakly expressed endogenous Notch in the adjacent cells, an NICD-responsive promoter, P TP1 , is activated [24] ( Supplementary Fig. 1a ). Under the control of P TP1 , the expression of an artificial transcriptional repressor, tTS, is induced. The induced tTS binds to a tTS-responsive promoter, P TetO , and then represses the expression of Delta, resulting in mutual transcriptional repression of Delta between adjacent cells ( Fig. 1a ). The expression levels of Delta and tTS were monitored by fluorescent reporter constructs joined by a self-cleaving 2A peptide [25] , Delta-2A-mCherry and tTS-2A-GFP. Thus, Delta-positive cells should exhibit red fluorescence, whereas Notch-active cells (that is, tTS-positive cells) should exhibit green fluorescence. However, cells engineered with the bTR circuit (hereafter called bTR cells) did not bifurcate into two distinct cell types but remained red (that is, a Delta-positive and tTS-negative state; Fig. 1b,c ), indicating that the bTR circuit does not meet conditions for cell-type bifurcation. 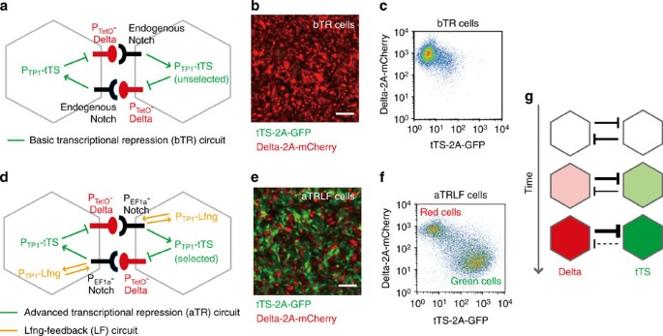Figure 1: Construction of lateral inhibition circuits for cell-type bifurcation in CHO cells. (a) A scheme for the bTR circuit. Binding of Delta to endogenous Notch between adjacent cells induces the transcription of the tTS repressor from the TP1 promoter, PTP1. Then, tTS represses the transcription of Delta from the TetO promoter, PTetO. (b) A typical image of a bTR cell clone. The entire cell population was Delta-positive and tTS-negative. Scale bar, 100 μm. (c) A unimodal distribution of the bTR cells. The cells were analysed by FACS for GFP and mCherry fluorescence. (d) A scheme for the aTRLF circuit, which comprises the aTR circuit and the LF circuit. In the aTR circuit, an exogenous Notch gene was introduced. In addition, cell clones that showed a higher induction level of tTS were selected. In the LF circuit, activation of Notch induces the transcription of Lfng from the PTP1, and Lfng in turn enhances the activation of Notch. An additional negative effect of Lfng on Delta was shown in this study. (e) A typical image of an aTRLF cell clone. The cell population contained Delta-positive cells and tTS-positive cells. Scale bar, 100 μm. (f) A bimodal distribution of the aTRLF cells. The cells were analysed by FACS for GFP and mCherry fluorescence. (g) A scheme for cell-type bifurcation between adjacent cells. Initially, two cells have similar expression levels of the components of the lateral inhibition circuit, such as Delta, tTS and Lfng. If a slight difference in these expression levels arises from noise, the difference is self-amplified by the lateral inhibition circuit. Figure 1: Construction of lateral inhibition circuits for cell-type bifurcation in CHO cells. ( a ) A scheme for the bTR circuit. Binding of Delta to endogenous Notch between adjacent cells induces the transcription of the tTS repressor from the TP1 promoter, P TP1 . Then, tTS represses the transcription of Delta from the TetO promoter, P TetO . ( b ) A typical image of a bTR cell clone. The entire cell population was Delta-positive and tTS-negative. Scale bar, 100 μm. ( c ) A unimodal distribution of the bTR cells. The cells were analysed by FACS for GFP and mCherry fluorescence. ( d ) A scheme for the aTRLF circuit, which comprises the aTR circuit and the LF circuit. In the aTR circuit, an exogenous Notch gene was introduced. In addition, cell clones that showed a higher induction level of tTS were selected. In the LF circuit, activation of Notch induces the transcription of Lfng from the P TP1 , and Lfng in turn enhances the activation of Notch. An additional negative effect of Lfng on Delta was shown in this study. ( e ) A typical image of an aTRLF cell clone. The cell population contained Delta-positive cells and tTS-positive cells. Scale bar, 100 μm. ( f ) A bimodal distribution of the aTRLF cells. The cells were analysed by FACS for GFP and mCherry fluorescence. ( g ) A scheme for cell-type bifurcation between adjacent cells. Initially, two cells have similar expression levels of the components of the lateral inhibition circuit, such as Delta, tTS and Lfng. If a slight difference in these expression levels arises from noise, the difference is self-amplified by the lateral inhibition circuit. Full size image Thus, we modified the bTR circuit and constructed an advanced transcriptional repression (aTR) circuit ( Fig. 1d , green arrows). To increase the amount of tTS that is induced on activation of Notch, we first introduced an exogenous Notch gene expressed under the control of a strong constitutive promoter, P EF1a , because overexpression of the exogenous Notch increased the P TP1 activity in a dose-dependent manner ( Supplementary Fig. 1b ). The expression level of P EF1a -Notch was roughly comparable to the Notch expression level in neural stem cells that are known to have a native lateral inhibition mechanism [3] , [12] , [13] , [14] ( Supplementary Fig. 1c ). Second, we selected a cell clone with a higher induction level of tTS. Considering the fact that more than 40 arbitrary fluorescence units (AFUs) of the tTS-2A-GFP signal are required to effectively repress the P TetO activity ( Supplementary Fig. 1d ), we selected cell clones where more than 100 AFU of tTS-2A-GFP were induced from the P TP1 ( Supplementary Fig. 1e ). To this end, the P TP1 -tTS-2A-GFP construct was introduced by an efficient transposon vector, piggyBac [26] , while other constructs were introduced by a lentiviral vector. In fact, those cell clones that passed the 100 AFU threshold were found to contain more than 10 copies of the P TP1 -tTS-2A-GFP construct, while containing only a single copy of the P EF1a -Notch and P TetO -Delta-2A-mCherry construct ( Supplementary Fig. 2 ). As a result of these improvements, a P TetO -luciferase reporter construct showed an 18-fold decrease on activation of Notch ( Supplementary Fig. 3a ). To further enhance the tTS induction and P TetO repression, we added a Lfng-feedback (LF) circuit ( Fig. 1d , yellow arrows). Lfng is a glycosyltransferase that glycosylates Notch and thereby enhances the binding of Notch to Delta [27] , [28] , [29] , [30] . In turn, the activation of Notch is known to induce the expression of Lfng [31] , [32] . To mimic the intracellular positive feedback relationship of Notch and Lfng in vivo , we introduced a P TP1 -Lfng construct. The P TP1 -Lfng construct then enhanced the P TP1 activity ( Supplementary Fig. 3b ), suggesting that the induction of Lfng expression by Notch and the enhancement of Notch activity by Lfng constitute an intracellular positive feedback loop. Thus, the combined genetic circuit of the aTR circuit and LF circuit was named an aTRLF circuit ( Fig. 1d ). Cell-type bifurcation among genetically identical cells Cells engineered with the aTRLF circuit (hereafter called aTRLF cells) spontaneously bifurcated into red cells (that is, Delta-positive and tTS-negative cells) and green cells (that is, Delta-negative and tTS-positive cells) ( Fig. 1e–g ). Importantly, the aTRLF cells showed a bimodal distribution ( Fig. 1f ). Yellow cells (that is, Delta-positive and tTS-positive cells) or colourless cells (that is, Delta-negative and tTS-negative cells) were very rare at the steady state ( Fig. 1e,f ). The expression of Delta was detected only in the red cell population, whereas that of tTS or Lfng was detected only in the green cell population ( Supplementary Fig. 3c ). Pharmacological inhibition of Delta–Notch signalling converted the bimodal distribution into a unimodal distribution and made all the cells red ( Supplementary Fig. 3d ), confirming that the formation of the bimodal distribution was mediated by the Delta–Notch signaling. These results suggest that the aTRLF circuit is bistable, whereas the bTR circuit is monostable. Similar unimodal distributions were obtained for other clones of bTR cells ( Supplementary Fig. 4a ), whereas similar bimodal distributions for other aTRLF cell clones ( Supplementary Fig. 4b ). It is noteworthy that the ratio of the red cells to green cells varied to some extent among the 30 aTRLF cell clones we isolated, and that a few aTRLF cell clones failed to show a clear bimodal distribution ( Supplementary Fig. 4b ). We used the aTRLF cell clones that showed a clear bimodal distribution for further analyses. Time-lapse imaging of proliferating aTRLF cells from a single cell revealed the cell-type bifurcation process in a single-cell colony ( Fig. 2a , Supplementary Fig. 5 and Supplementary Movie 1 ). Red cells dominated as long as the cell number was low. When the cell number reached ~100 cells, some cells started to make a transition to the green state, eventually resulting in a salt-and-pepper pattern of the red cells and green cells ( Fig. 2a and Supplementary Fig. 5b ). These results indicate that the aTRLF circuit has the ability to cause cell-type bifurcation among a genetically identical cell population. 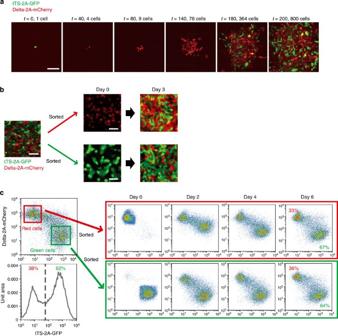Figure 2: Robustness of the cell-type ratio in cell population. (a) Time-lapse imaging of cell-type bifurcation in an aTRLF cell colony. A single aTRLF cell, which happened to be green, was seeded. The cell proliferated and then changed the colour according to the total cell number. Scale bar, 100 μm. SeeSupplementary Movie 1. (b,c) The aTRLF cells were sorted into the red cell fraction and green cell fraction. The red cells and green cells were seeded separately at the same cell densities. (b) Three days after sorting, green cells were detected in the sorted red cell fraction (upper), whereas red cells were detected in the sorted green cell fraction (lower). Scale bar, 50 μm. SeeSupplementary Movie 2. (c) The sorted cells were re-seeded and analysed by FACS every other day. Six days after sorting, the original cell-type ratio was reproduced in each fraction culture. The ratio of red cells to green cells was defined by the broken grey line. Figure 2: Robustness of the cell-type ratio in cell population. ( a ) Time-lapse imaging of cell-type bifurcation in an aTRLF cell colony. A single aTRLF cell, which happened to be green, was seeded. The cell proliferated and then changed the colour according to the total cell number. Scale bar, 100 μm. See Supplementary Movie 1 . ( b , c ) The aTRLF cells were sorted into the red cell fraction and green cell fraction. The red cells and green cells were seeded separately at the same cell densities. ( b ) Three days after sorting, green cells were detected in the sorted red cell fraction (upper), whereas red cells were detected in the sorted green cell fraction (lower). Scale bar, 50 μm. See Supplementary Movie 2 . ( c ) The sorted cells were re-seeded and analysed by FACS every other day. Six days after sorting, the original cell-type ratio was reproduced in each fraction culture. The ratio of red cells to green cells was defined by the broken grey line. Full size image Robustness of the cell-type ratio in cell population Using the aTRLF cells, we investigated whether the ratio of red cells to green cells is reproducible, or robust, as robustness of cell-type ratios should be pivotal for the development of multicellular organisms. The red cell fraction and green cell fraction were sorted and cultured separately ( Fig. 2b,c ). During 3 days of culture, a portion of the sorted red cells made a transition to the green state, and a portion of the sorted green cells made a transition to the red state ( Fig. 2b and Supplementary Movie 2 ). Remarkably, after 6 days a bimodal distribution was fully reproduced in each fraction culture and the cell-type ratios in both cultures were quite similar to each other ( Fig. 2c and Supplementary Fig. 6 ). In a typical aTRLF cell clone that showed a clear bimodal distribution, the cell-type ratio before sorting was red:green=38:62 and the recovered cell-type ratios were red:green=33:67 and 36:64 ( Fig. 2c ). These results indicate that the lateral inhibition mechanism between adjacent cells governs the ratio of two cell types at the cell-population level, and that the cell-type ratio is robust against temporal perturbation. Static equilibrium of the cell-type ratio A robust cell-type ratio at the steady state indicates two possibilities—(1) static equilibrium: at the steady state, the red cells remain red and the green cells remain green; (2) dynamic equilibrium: although the cell-type ratio remains constant, transitions are occurring from the red state to the green state, and vice versa . To discriminate between the two possibilities, we labelled the sorted red cells with a far-red fluorescent marker and mixed the labelled red cells and unlabelled green cells at different ratios ( Fig. 3a ). Whereas the labelled red cells showed transitions to the green state when the initial mix ratio (red:green) was 10:0, most of the labelled red cells remained red when the mix ratio was 4:6 or 2:8 ( Fig. 3a , see the upper right fraction in each fluorescence-activated cellsorting (FACS) plot). Namely, the transition rate from the red state to the green state showed a correlation with the mix ratio of red cells ( Fig. 3b , blue bars). Likewise, the transition rate from the green state to the red state showed a correlation with the mix ratio of green cells ( Fig. 3b , pink bars). The total transition rate was at a minimum when the mix ratio was 4:6 ( Fig. 3b ), suggesting that the cells tend not to change their colours when the mix ratio is close to the cell-type ratio at the steady state (according to Fig. 2c , red:green=38:62). Essentially, the same results were obtained when the green cells were labelled instead of the red cells ( Supplementary Fig. 7 ). These results support the static equilibrium model at the steady state, where most, if not all, of the cells tend to remain in their present colour states ( Fig. 3c ). 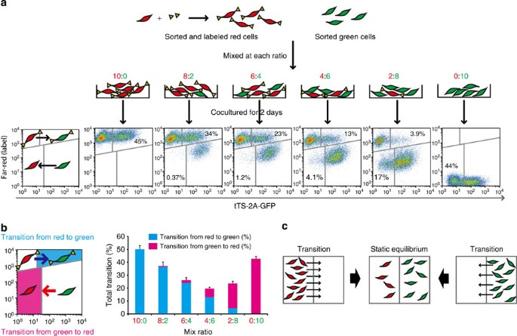Figure 3: Static equilibrium of the cell-type ratio. (a) The aTRLF cells were sorted by their colours using FACS. The sorted red cells were labelled with a far-red fluorescent marker. The labelled red cells and unlabelled green cells were mixed and cocultured at the indicated ratios. Two days later, the cells were analysed by FACS for GFP and far-red fluorescence. (b) Quantification of the transition rates shown ina. The labelled green cells indicate transitions from the red state to the green state, whereas the unlabelled red cells indicate transitions from the green state to the red state. Data are means+s.e.m. (n=3). (c) A scheme for static equilibrium. When the mix ratio is far from the cell-type ratio at the steady state (according toFig. 2c, red:green=38:62), the cells change their colours (left and right). Once the cell-type ratio at the steady state is achieved, the cells no longer change their colours (middle). Figure 3: Static equilibrium of the cell-type ratio. ( a ) The aTRLF cells were sorted by their colours using FACS. The sorted red cells were labelled with a far-red fluorescent marker. The labelled red cells and unlabelled green cells were mixed and cocultured at the indicated ratios. Two days later, the cells were analysed by FACS for GFP and far-red fluorescence. ( b ) Quantification of the transition rates shown in a . The labelled green cells indicate transitions from the red state to the green state, whereas the unlabelled red cells indicate transitions from the green state to the red state. Data are means+s.e.m. ( n =3). ( c ) A scheme for static equilibrium. When the mix ratio is far from the cell-type ratio at the steady state (according to Fig. 2c , red:green=38:62), the cells change their colours (left and right). Once the cell-type ratio at the steady state is achieved, the cells no longer change their colours (middle). Full size image Temporal dynamics of cell-type bifurcation Next, to investigate the dynamics of cell-type bifurcation, we created a lateral inhibition circuit with faster fluorescent reporters by fusing the protein destabilizing signal sequence, d2PEST, to green fluorescent protein (GFP) and mCherry ( Fig. 4a ). The half-life of d2PEST is reported to be 2 h (ref. 33 ), which is roughly comparable to the half-life of Delta (2.5 h) or that of tTS (0.5 h; Supplementary Fig. 8 ). As expected, the aTRLF cells with the d2PEST reporters (hereafter called aTRLFd2 cells) showed a bimodal distribution at the steady state ( Fig. 4b ). When aTRLFd2 cells were forced into the red state by the pharmacological inhibition of Delta–Notch signalling and then released from the inhibition, we observed a yellow cell population that was making a transition to the green state ( Fig. 4c,d and Supplementary Movie 3 ). On the other hand, when the cell-type ratio was at the steady state, most cells did not change their colours even after cell divisions ( Fig. 4e and Supplementary Movie 3 ). This is probably because the CHO cells quickly intermingle after cell divisions and meet multiple new neighbours, whose red/green ratio is roughly constant at the steady state. In such a situation, it should be easier for the cells to remain in the present colour state. We occasionally detected, however, colour flipping events ( Fig. 4e , arrowheads), probably because the cell-type ratio of the neighbouring cells may deviate from the constant ratio accidentally and locally, and then the surrounded cell needs to make a transition to the other colour state. These results are consistent with our cell-labelling experiments ( Fig. 3 ). 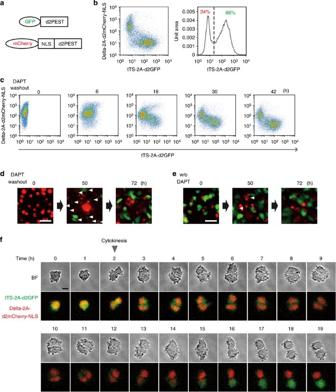Figure 4: Temporal dynamics of cell-type bifurcation. (a) A scheme for faster fluorescent reporters. A d2PEST sequence was fused to GFP and mCherry to make their half-lives shorter. A nuclear localization signal (NLS) was also fused to mCherry to make microscopy observation easier. (b) The aTRLFd2 cells were analysed by FACS. (c,d) The aTRLFd2 cells were treated with 3 μM DAPT for 2 days. After DAPT was washed out, the cells were seeded at a density of 8 × 105cells per 35-mm dish. (c) The cells released from the DAPT treatment were analysed by FACS at indicated time points. (d) Time-lapse imaging of the cells released from the DAPT treatment. Arrowheads indicate the cells that are changing their colours. Scale bar, 50 μm. SeeSupplementary Movie 3, left. (e) Time-lapse imaging of the aTRLFd2 cells at the steady state. The aTRLFd2 cells were seeded at a density of 8 × 105cells per 35-mm dish. Arrowheads indicate occasional colour flipping events. Scale bar, 100 μm. SeeSupplementary Movie 3, right. (e) Time-lapse imaging of cell-type bifurcation between two daughter aTRLFd2 cells. A mother cell was seeded on micropatterned cultureware, where a cell-substratum attachment area is a 25-μm square. Scale bar, 10 μm. SeeSupplementary Movie 4. Figure 4: Temporal dynamics of cell-type bifurcation. ( a ) A scheme for faster fluorescent reporters. A d2PEST sequence was fused to GFP and mCherry to make their half-lives shorter. A nuclear localization signal (NLS) was also fused to mCherry to make microscopy observation easier. ( b ) The aTRLFd2 cells were analysed by FACS. ( c , d ) The aTRLFd2 cells were treated with 3 μM DAPT for 2 days. After DAPT was washed out, the cells were seeded at a density of 8 × 10 5 cells per 35-mm dish. ( c ) The cells released from the DAPT treatment were analysed by FACS at indicated time points. ( d ) Time-lapse imaging of the cells released from the DAPT treatment. Arrowheads indicate the cells that are changing their colours. Scale bar, 50 μm. See Supplementary Movie 3 , left. ( e ) Time-lapse imaging of the aTRLFd2 cells at the steady state. The aTRLFd2 cells were seeded at a density of 8 × 10 5 cells per 35-mm dish. Arrowheads indicate occasional colour flipping events. Scale bar, 100 μm. See Supplementary Movie 3 , right. ( e ) Time-lapse imaging of cell-type bifurcation between two daughter aTRLFd2 cells. A mother cell was seeded on micropatterned cultureware, where a cell-substratum attachment area is a 25-μm square. Scale bar, 10 μm. See Supplementary Movie 4 . Full size image Furthermore, using the aTRLFd2 cells we investigated whether our lateral inhibition circuit is able to break ‘symmetry’ even between two daughter cells ( Fig. 4f ). As daughter cells are born from the same mother cell, they are expected to initially possess a similar gene expression profile. We enhanced cell–cell contacts between adjacent cells by using micropatterned cultureware, where the cell–substratum attachment area is restricted (a 25-μm square) such that the cells within the area cannot separate from each other. Under the condition, we successfully detected symmetry-breaking events: after a mother aTRLFd2 cell divided into two daughter cells, the two cells went through a ‘battling phase’ in which their colours were not decisive, and then one daughter cell became bright red, whereas the other cell became bright green ( Fig. 4f , Supplementary Fig. 9 and Supplementary Movie 4 ). These results suggest that the aTRLF circuit has the ability to amplify a small initial difference between two cells. The cell-type ratio is adjustable by cell–cell attachment Thus far, we have shown that the cell-type ratio is constant and robust against perturbation ( Figs 2 and 3 ). We then investigated what alters the cell-type ratio, because the ratio regulated by lateral inhibition often varies across species and tissues. As the time-lapse imaging of aTRLF cells suggested a relationship of the total cell number and the cell-type ratio ( Fig. 2a ), we altered the cell seeding density ( Fig. 5a,b and Supplementary Fig. 10a ). When the cells were seeded at a high density, the distribution of the cell population was bimodal and the ratio of red cells to green cells was 32:68 ( Fig. 5b , 1.5 × 10 6 cells). In contrast, when the cell-seeding density was lower, the distribution became unimodal and the proportion of red cells dramatically increased. At the lowest cell density we examined, the proportion of red cells exceeded 90% ( Fig. 5b , 5 × 10 3 cells). A plausible explanation for the ‘density effect’ on the cell-type ratio is that when cell density is low, direct cell–cell contacts are less frequent and, therefore, binding of Delta to Notch between adjacent cells should be less frequent. Without the Delta–Notch binding, P TP1 -tTS-2A-GFP is not activated and P TetO -Delta-2A-mCherry is not repressed. As a result, the red cells should become dominant. In support of this hypothesis, pharmacological inhibition of Delta–Notch signalling produced a very similar transition of the cell-type ratio ( Supplementary Fig. 10b,c ; compare Fig. 5b with Supplementary Fig. 10c ). 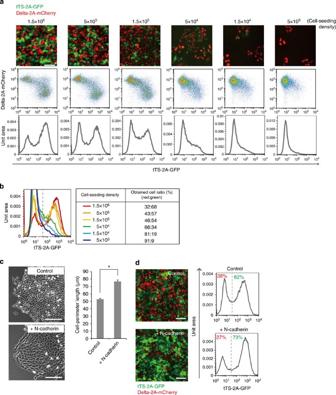Figure 5: The cell-type ratio is adjustable by the degree of cell–cell attachment. (a) Density effects on the cell-type ratio. The aTRLF cells were seeded at the indicated densities (cells per 35-mm dish). Two days later, the cells were re-seeded at the same densities to make sure that the system reaches a steady state. Two more days later, the images were taken and the cells were analysed by FACS. Scale bar, 100 μm. (b) The relationship between the cell density and the cell-type ratio. Quantification of the cell-type ratio of the FACS plots shown in (a). (c) Typical morphology of a cell colony of an aTRLF cell clone and that of the corresponding cell clone with N-cadherin overexpression (left). Scale bar, 100 μm. Quantification of the length of cell perimeter (right). Data are means+s.e.m. (n=30). *P<0.01 (Welch’st-test). (d) The aTRLF cells without or with N-cadherin overexpression were seeded at a density of 8 × 105cells per 35-mm dish. Two days later, the cells were re-seeded. Two more days later, the images were taken and the cell-type ratios were analysed by FACS. Scale bar, 100 μm. Figure 5: The cell-type ratio is adjustable by the degree of cell–cell attachment. ( a ) Density effects on the cell-type ratio. The aTRLF cells were seeded at the indicated densities (cells per 35-mm dish). Two days later, the cells were re-seeded at the same densities to make sure that the system reaches a steady state. Two more days later, the images were taken and the cells were analysed by FACS. Scale bar, 100 μm. ( b ) The relationship between the cell density and the cell-type ratio. Quantification of the cell-type ratio of the FACS plots shown in ( a ). ( c ) Typical morphology of a cell colony of an aTRLF cell clone and that of the corresponding cell clone with N-cadherin overexpression (left). Scale bar, 100 μm. Quantification of the length of cell perimeter (right). Data are means+s.e.m. ( n =30). * P <0.01 (Welch’s t -test). ( d ) The aTRLF cells without or with N-cadherin overexpression were seeded at a density of 8 × 10 5 cells per 35-mm dish. Two days later, the cells were re-seeded. Two more days later, the images were taken and the cell-type ratios were analysed by FACS. Scale bar, 100 μm. Full size image Next, we attempted to do the opposite: increase the proportion of green cells. To enhance cell–cell adhesion, we introduced an adhesion molecule, N-cadherin, into the aTRLF cells ( Supplementary Fig. 11a ). Overexpression of N-cadherin under a constitutive promoter, P CAG [34] , changed CHO cell morphology; the cells became less elongated and the colony appeared more tightly packed ( Fig. 5c ). The N-cadherin overexpression increased the proportion of green cells from 62% to 73% ( Fig. 5d and Supplementary Fig. 11b ). Essentially, the same results were obtained when N-cadherin was introduced into other aTRLF cell clones ( Supplementary Fig. 11c ). We noticed that the cell perimeter was longer in the N-cadherin-expressing cells ( Fig. 5c , right). In addition, the N-cadherin-expressing aTRLF cells tended to cluster together even at lower cell densities, while the control aTRLF cells tended to disperse ( Supplementary Fig. 11d and Supplementary Movie 5 ). Thus, N-cadherin may contribute to the increased proportion of green cells (that is, Notch-active cells) by increasing the degree of cell–cell attachment and therefore enhancing the frequency of Delta–Notch signalling. These results indicate that the cell-type ratio in our system is finely adjustable by the degree of cell–cell attachment that is affected by the cell density and cell–cell adhesion. Effects of the LF circuit on the cell-type ratio As another means to alter the cell-type ratio, we focused on the architecture of the lateral inhibition circuit, especially on the role of the LF circuit. We first attempted to clarify the effect of Lfng on Delta–Notch signalling, because Lfng has been reported to act as either a positive or negative modulator of the Delta–Notch signalling, depending on the context [27] , [28] , [29] , [30] , [32] , [35] . A series of coculture experiments revealed that when Lfng was expressed only in ‘Receptor cells’, which have Notch and its reporter construct, the presence of Lfng increased the reporter activity ( Fig. 6a and Supplementary Fig. 12a ). In contrast, when Lfng was expressed also in ‘Ligand cells’, which continuously produce large amounts of Delta, the presence of Lfng decreased the reporter activity of Receptor cells ( Fig. 6b and Supplementary Fig. 12b ). These results indicate that Lfng has a positive effect on the Notch receptor and a negative effect on the Delta ligand in our system ( Fig. 6c ). Thus, not only the aTR circuit but also the LF circuit serves as a lateral inhibition mechanism between adjacent cells ( Fig. 6c ). In addition, the negative effect of Lfng on Delta was dependent on the expression of Notch in the same Ligand cells ( Supplementary Fig. 12b ) and the positive effect of Lfng on Notch was more prominent in the presence of the Notch expression in the Ligand cells ( Supplementary Fig. 12a ), suggesting involvement of cis -inhibition (see Discussion). 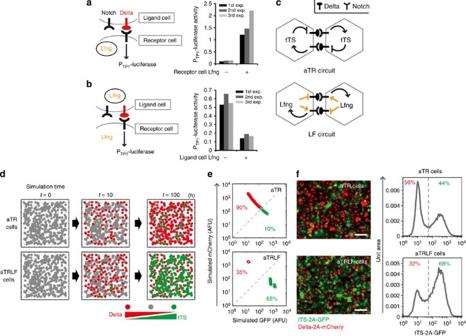Figure 6: The LF circuit alters the cell-type ratio. (a) A positive effect of Lfng on the Notch receptor. CHO cells that have PEF1a-Notch, PTP1-luciferase and PCMV-Lfng constructs (Receptor cells) were cocultured with CHO cells that have PSV40-Delta and PEF1a-Notch constructs (Ligand cells) at a ratio of 1:9. The luciferase activities were measured in the absence or presence of Lfng in the Receptor cells. (b) A negative effect of Lfng on the Delta ligand. CHO cells that have PEF1a-Notch, PTP1-luciferase and PCMV-Lfng constructs (Receptor cells) were cocultured with CHO cells that have PSV40-Delta, PEF1a-Notch and PCMV-Lfng constructs (Ligand cells). The luciferase activities were measured in the absence or the presence of Lfng in the Ligand cells. (c) A scheme for the aTR circuit and a revised scheme for the LF circuit. Lfng has a positive effect on Notch and a negative effect on Delta. Both the aTR circuit and LF circuit constitute intercellular (double-negative) positive feedback loops. (d) Numerical simulations of the mathematical models for the aTR cells and aTRLF cells, with 400 cells in an 8 × 8 grid and a random cell arrangement. The cells within 0.5 radius were considered as the adjacent cells. Hill coefficientn=2. (e) Simulated cell-type ratios shown ind,t=100 h. (f) Experimental verification of ratio alteration by the LF circuit. A cell clone that has only the aTR circuit (aTR cells) was compared with the corresponding cell clone that has both the aTR and LF circuits (aTRLF cells). Scale bar, 100 μm. Figure 6: The LF circuit alters the cell-type ratio. ( a ) A positive effect of Lfng on the Notch receptor. CHO cells that have P EF1a -Notch, P TP1 -luciferase and P CMV -Lfng constructs (Receptor cells) were cocultured with CHO cells that have P SV40 -Delta and P EF1a -Notch constructs (Ligand cells) at a ratio of 1:9. The luciferase activities were measured in the absence or presence of Lfng in the Receptor cells. ( b ) A negative effect of Lfng on the Delta ligand. CHO cells that have P EF1a -Notch, P TP1 -luciferase and P CMV -Lfng constructs (Receptor cells) were cocultured with CHO cells that have P SV40 -Delta, P EF1a -Notch and P CMV -Lfng constructs (Ligand cells). The luciferase activities were measured in the absence or the presence of Lfng in the Ligand cells. ( c ) A scheme for the aTR circuit and a revised scheme for the LF circuit. Lfng has a positive effect on Notch and a negative effect on Delta. Both the aTR circuit and LF circuit constitute intercellular (double-negative) positive feedback loops. ( d ) Numerical simulations of the mathematical models for the aTR cells and aTRLF cells, with 400 cells in an 8 × 8 grid and a random cell arrangement. The cells within 0.5 radius were considered as the adjacent cells. Hill coefficient n =2. ( e ) Simulated cell-type ratios shown in d , t =100 h. ( f ) Experimental verification of ratio alteration by the LF circuit. A cell clone that has only the aTR circuit (aTR cells) was compared with the corresponding cell clone that has both the aTR and LF circuits (aTRLF cells). Scale bar, 100 μm. Full size image We then built a mathematical model that incorporates the dual effects of Lfng (see Methods; Supplementary Table 1 ), to investigate how the LF circuit affects the cell-type ratio. Numeric simulations of the mathematical model predicted that the proportion of green cells in the aTRLF cells should be higher than that in the cells engineered only with the aTR circuit (hereafter called aTR cells; Fig. 6d,e ). To test this predication, we compared an aTR cell clone with the corresponding clone that had been further engineered with the LF circuit (that is, an aTRLF cell clone). The aTR cells showed a bimodal distribution ( Fig. 6f , upper), suggesting that the aTR circuit is also bistable. Importantly, the proportion of green cells in the aTRLF cells (68%) was substantially higher than that in the aTR cells (44%; Fig. 6f ), in accordance with our prediction. Essentially, the same results were obtained when the LF circuit was added to another aTR cell clone ( Supplementary Fig. 13a ). An intuitive explanation of the ratio alteration by the LF circuit is that as the aTRLF circuit contains two intercellular (double-negative) positive feedback loops (that is, the aTR circuit and LF circuit, see Fig. 6c ), the aTRLF circuit should be able to create a stable difference among adjacent cells with an increased frequency. Note that the frequency of cell-type bifurcation is reflected in the proportion of green cells; without cell-type bifurcation, the cells remain red (see Fig. 5a , 5 × 10 3 cells and Supplementary Fig. 3d ). Thus, addition of the LF circuit should increase the frequency of cell-type bifurcation and therefore increase the proportion of green cells. In fact, knockout or knockdown of Lfng has been reported to decrease the proportion of Notch-active cells (represented by the green cells in our study) in the developing vertebrate nervous system [36] , [37] . In addition, bifurcation diagrams of the mathematical model indicated that addition of the LF circuit expands the parameter space for bistability ( Supplementary Fig. 13b ). Namely, the aTRLF circuit should attain bistability more easily than the aTR circuit. In accordance with the prediction, the aTRLF cells tended to show clearer separation of the two cell types in the bimodal distribution as compared with the aTR cells ( Supplementary Fig. 13c ). Cell-type bifurcation without the aTR circuit Although lateral inhibition usually refers to mutual transcriptional repression of Delta between adjacent cells (represented by the aTR circuit in our study), our results indicated that the LF circuit also serves as a lateral inhibition mechanism ( Fig. 6c ). Thus, we assessed whether the LF circuit alone is capable of cell-type bifurcation. To this end, the aTR circuit was specifically blocked by the tTS inhibitor, Doxycycline (Dox; Fig. 7a ). Our mathematical model predicted that the LF circuit should be able to attain bistability even without the aTR circuit ( Fig. 7b ). In accordance with this prediction, the aTRLF cells showed a bimodal distribution even in the presence of Dox, whereas the aTR cells did not ( Fig. 7c and Supplementary Fig. 13d ). In the Dox-treated aTRLF cells, the expression of Lfng was detected only in the GFP-positive (that is, Notch-active) cell population ( Fig. 7d ). These results suggest importance of the LF circuit in cell-type bifurcation. 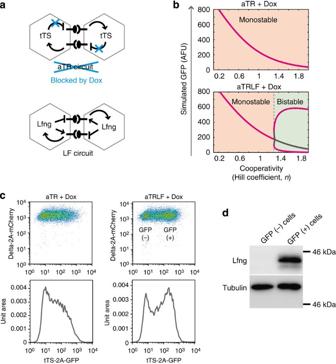Figure 7: Cell-type bifurcation without the aTR circuit. A scheme for inhibition of the aTR circuit with Dox. Dox inhibits the function of tTS. The LF circuit remains intact. (b) Bifurcation diagrams of the mathematical models for the aTR circuit and aTRLF circuit in the presence of Dox. (c) The aTR cells and aTRLF cells were treated with 30 ng ml−1Dox. Two days later, the cells were re-seeded and again treated with Dox to make sure that the system reaches a steady state. Two more days later, the cells were analysed by FACS. The aTRLF cells bifurcated into the GFP-negative cells and GFP-positive cells. (d) The GFP-negative aTRLF cells and GFP-positive aTRLF cells shown inc, the upper right panel, were sorted by FACS. The expression level of Lfng was measured in each cell fraction by immunoblotting. The control, Tubulin, was run on a different gel. Figure 7: Cell-type bifurcation without the aTR circuit. A scheme for inhibition of the aTR circuit with Dox. Dox inhibits the function of tTS. The LF circuit remains intact. ( b ) Bifurcation diagrams of the mathematical models for the aTR circuit and aTRLF circuit in the presence of Dox. ( c ) The aTR cells and aTRLF cells were treated with 30 ng ml −1 Dox. Two days later, the cells were re-seeded and again treated with Dox to make sure that the system reaches a steady state. Two more days later, the cells were analysed by FACS. The aTRLF cells bifurcated into the GFP-negative cells and GFP-positive cells. ( d ) The GFP-negative aTRLF cells and GFP-positive aTRLF cells shown in c , the upper right panel, were sorted by FACS. The expression level of Lfng was measured in each cell fraction by immunoblotting. The control, Tubulin, was run on a different gel. Full size image We previously constructed a genetic circuit for mutual activation of Delta–Notch signalling between adjacent cells to demonstrate signal propagation [23] . In this study, on the other hand, we aimed to construct a genetic circuit for lateral inhibition between adjacent cells that gives rise to cell-type bifurcation. Among different types of lateral inhibition circuits we constructed, the aTR circuit, LF circuit and aTRLF circuit made adjacent cells spontaneously bifurcate into two distinct cell types, while the bTR circuit was not sufficient for the cell-type bifurcation. The frequency of cell-type bifurcation (that is, the proportion of green cells) was highest in the aTRLF cells. The aTRLF circuit even showed the ability to amplify a small initial difference between two daughter cells. Although a bistable system usually requires nonlinearity that is derived from cooperative regulatory processes in the genetic circuit, our mathematical model showed that the combination of the aTR circuit and LF circuit enables the aTRLF circuit to attain bistability without assuming any cooperativity (that is, Hill coefficient=1, or lower) in the transcriptional regulations of P TP1 and P TetO ( Supplementary Fig. 13b ). In fact, activation of P TP1 has been reported not to have significant cooperativity [38] and repression of P TetO did not show significant cooperativity in our measurement ( Supplementary Fig. 1d ). Thus, the combination of the aTR circuit and LF circuit should be beneficial to increase the certainty of cell-type bifurcation. The sufficiency of the LF circuit alone for cell-type bifurcation was surprising, because lateral inhibition usually refers to the transcriptional repression of Delta (that is, aTR circuit). We have found that Lfng has both positive and negative effects on Delta–Notch signalling in our system. Although the molecular mechanisms by which Lfng exerts the dual effects are unclear, the negative effect of Lfng on Delta was dependent on the expression of Notch in the same cells ( Supplementary Fig. 12b ). In addition, the two cell types bifurcated by the LF circuit did not differ in the transcription level of Delta ( Fig. 7c , see the Delta-2A-mCherry fluorescence) but differed in the activation level of Notch ( Fig. 7c , see the tTS-2A-GFP fluorescence). Thus, our working hypothesis is that the negative effect of Lfng may be mediated by cis -inhibition ( Supplementary Fig. 14a ), which is caused by deprivation of Delta through the cis -binding of Notch to Delta within the same cell [11] , [38] , [39] . Lfng may glycosylate Notch and thereby enhance the binding of Notch to Delta [29] , [30] both in trans (that is, between the adjacent cells) and in cis (that is, within the same cell). The enhancement of trans -binding may cause the positive effect on the Notch receptor, whereas that of cis -binding may cause the negative effect on the Delta ligand. Lateral inhibition controlled by Delta–Notch signalling is a mechanism that works locally between adjacent cells. In this study, however, the entire cell population engineered with the aTRLF circuit spontaneously bifurcated into two cell types with a particular ratio. Importantly, the cell-type ratio was robust: the original ratio was spontaneously reproduced even after the two cell types were separated and mixed at different ratios. Thus, the lateral inhibition mechanism has the ability to robustly maintain the cell-type ratio in a cell population ( Supplementary Fig. 14b ). The robust ratio regulation may be able to guarantee the appropriate balance of distinct cell types in tissues even when the tissue homeostasis is temporally disturbed by injuries or biological noise [40] , [41] . The cell-type ratio regulated by lateral inhibition varies widely across species and tissues. The ratio of hair cells to supporting cells in the chick inner ear is ~1:2 (ref. 19 ), while the ratio of bristle precursor cells to surrounding epithelial cells in Drosophila is ~1:30 (ref. 10 ). Long-range activation of Delta–Notch signalling through filopodial contacts has been proposed to explain the different cell-type ratio [10] . Inhibition of Delta–Notch signalling has been shown to alter the ratio of secretory cells to absorptive cells in the mouse intestine, whose normal ratio is ~1:9 (refs 16 , 42 ). In this study, we inquired whether other mechanisms would affect the cell-type ratio. We have shown that the cell-type ratio varies according to the degree of cell–cell attachment and the architecture of the genetic circuit. The proportion of green cells (that is, Notch-active cells) increased in proportion to the higher cell density and the stronger cell–cell adhesion. The LF circuit shifted the cell-type ratio to more Notch-active cells. In good agreement with our results, a knockout mouse of Lfng has been reported to show less Hes1-positive cells (that is, Notch-active cells) and more Ngn2-positive cells (that is, Delta-positive cells) in the developing nervous system [36] . Finally, the lateral inhibition circuit described in this study has a potential to recapitulate two other developmentally important phenomena: regular cell pattern formation and synchronized oscillation. Although the spatial arrangement of red cells and green cells shown in this study appeared random, the lateral inhibition mechanism is known to create a more regular salt-and-pepper pattern in several epithelial cell tissues, such as the inner ear [1] , [19] , [20] , [39] . In fact, our numerical simulation of the aTRLF model with a hexagonal cell arrangement resulted in a regular salt-and-pepper pattern ( Supplementary Fig. 14c ). On the other hand, the lateral inhibition mechanism is also known to regulate synchronized oscillation in segmentation clock [43] , [44] . Thus, the next challenge will be reconstituting a regular salt-and-pepper pattern as well as synchronized oscillation by using the lateral inhibition circuit to understand these self-organization mechanisms of development. DNA constructs The genetic constructs used in this study are listed in Supplementary Table 2 . Each promoter and gene were subcloned into pDONR to construct entry vectors according to the manufacturer’s protocol (Invitrogen). These entry clones were recombined with pLenti6.3 (Invitrogen) or piggyBac vector, using the Multisite Gateway technology (Invitrogen) [23] . Culture protocols CHO cells, provided by the RIKEN BRC through the National Bio-Resource Project of the MEXT, Japan, were maintained in DMEM/F12 medium containing 10% fetal bovine serum at 37 °C with 5% CO 2 . Mouse neural stem cells were purchased from R&D Systems. Creation of stable cell clones Viruses for each pLenti construct were created according to the manufacturer’s protocols (Invitrogen). CHO cells were infected with the viruses and maintained in the basal medium plus 10 μg ml −1 blasticidin, 1 μg ml −1 puromycin, 200 μg ml −1 hygromycin or 50 μg ml −1 G418 for the selection of drug-resistant clones [23] . CHO cells were also transfected with the piggyBa c construct and piggyBac transposase plasmid [26] . To construct the aTRLF circuit, the P EF1a -Notch construct was first introduced by lentiviruses and one cell clone that showed high Notch expression was isolated by limiting dilution. Next, the P TP1 -tTS-2A-GFP construct was introduced by piggyBac and the cells that showed a high induction rate of GFP (>100 AFU) on Notch activation were sorted by FACS. This step is the most important criterion in our clone screening. In fact, <5% cells passed this criterion. Finally, the P TetO -Delta-2A-mCherry and P TP1 -Lfng constructs were introduced by lentiviruses and cell clones were isolated by limiting dilution. Luciferase reporter assay For real-time luciferase assays, CHO cells engineered with each genetic construct were cocultured with Ligand cells at a ratio of 1:9 at a total density of 1 × 10 6 cells per 35-mm dish. Four hours later, luciferase substrate D -luciferin (0.1 mM) was added to the culture medium. Luciferase activity was recorded once every hour using Kronos Dio Luminometer (Atto). For non-real-time luciferase assays, the cells were cocultured with Ligand cells at a ratio of 1:9 at a density of 3 × 10 5 cells per well on a 12-well plate. After 40 h of coculture, luciferase activity was measured using a luciferase reporter assay system (Promega). Image and data analysis The cells were seeded at a density of 1 × 10 6 cells per 35-mm dish unless indicated otherwise. Two days later, the cells were re-seeded at the same densities to make sure that the system reaches a steady state. Two more days later, the cells were fixed with 3.7% formaldehyde and images were taken with Axio Observer A1 (Carl Zeiss) or IX73 (Olympus). Time-lapse imaging was performed with an incubator microscope system, LCV110 (Olympus). Data collection and analysis were performed with MetaMorph software (Molecular Devices). To enhance cell–cell contacts between daughter cells, cells were seeded on micropatterned cultureware, CytoGraph (DNP). FACS analysis and cell sorting For FACS analyses, the cells were seeded at a density of 1 × 10 6 cells per 35-mm dish unless indicated otherwise. Two days later, the cells were re-seeded at the same densities to make sure that the system reaches a steady state. Two more days later, the cells were quantified with JSAN (Bay bioscience) or FACSCalibur (BD) and analysed with FlowJo software. Cell sorting was performed with JSAN. The sorted mCherry-positive cells and GFP-positive cells were seeded separately at a density of 6 × 10 5 cells per 35-mm dish for time-lapse imaging and at a density of 4 × 10 5 cells per well on a 12-well plate for FACS analyses. For immunoblotting, 1 × 10 5 cells were sorted. Cell labelling and transition assessment The sorted cells were labelled with a far-red fluorescent marker, CellVue Maroon (POL), according to the manufacturer’s protocols. The labelled and unlabelled cells were cocultured at a density of 1.5 × 10 5 cells per well on a 24-well plate. Two days later, the cells were analysed by FACSCalibur or JSAN for GFP and far-red fluorescence. Immunoblotting Immunoblotting was performed by means of standard protocols. The blot was probed with rabbit anti-Myc (A14, Santa Cruz; 1/2,000), mouse anti-α-Tubulin (DM1A, Sigma; 1/20,000), goat anti-Delta (C-20, Santa Cruz; 1/2,000), rat anti-N-cadherin (NCD-2, gift from M. Takeichi; 1/1,000), rabbit anti-Tet-Repressor (TET01, MoBiTec; 1/2,000), or mouse anti-V5 antibody (46-0705, Invitrogen; 1/2,000). Original scans of immunoblottings are shown in Supplementary Fig. 15 . Southern blotting Southern blotting was performed according to the DIG Application Manual for Filter Hybridization (Roche) using the PCR DIG Probe Synthesis kit (Roche). The probe sequences are available in Supplementary Table 2 . Quantittive RT–PCR Total RNA was extracted with the RNeasy kit (Qiagen) and reverse transcribed with the QuantiTect Reverse Transcription kit (Qiagen). Real-time PCR was performed using LightCycler 480 II (Roche). The measured value was normalized to glyceraldehyde 3-phosphate dehydrogenase. Primers were designed in the messenger RNA sequence where the parts of the sequences are identical between mouse and hamster. The primer sequences are listed in Supplementary Table 2 . Degradation assay CHO cells engineered with each genetic construct were treated with cycloheximide (20 μg ml −1 ). The cells were frozen in liquid nitrogen at the indicated time points. Cell extracts were resolved by immunoblotting. Curve fitting was performed with Excel. Models We constructed simple mathematical models that represented the lateral inhibition circuits. 1. Model for aTR cells: 2. Model for aTRLF cells: The variables are N (Notch), G (glycosylated Notch), D (Delta), S (released NICD), R (tTS repressor), L (Lfng), F (GFP) and C (mCherry). The cis -inhibition model developed by Sprinzak et al. [39] was used as a reference of the model for aTR cells. Then, the effect of the LF circuit was added to construct the model for aTRLF cells. The expression of Lfng is induced by the same promoter as tTS (equation (12)). The induced Lfng gylcosylates Notch (equations (7 and 8)). The binding of glycosylated Notch to Delta (both in trans and in cis ) is k G -fold stronger than that of non-glycosylated Notch (equations (8, 9 and 10)). The parameter values are listed in Supplementary Table 1 . The symbol ‹› denotes the sum of the expression levels in adjacent cells divided by 6. Namely, where j and j′ are the indices of each cell and its adjacent cells, respectively. In the two cell models ( Fig. 7b and Supplementary Fig. 13b ), the ‘adjacent’ cell means the other cell. In the multiple cell models with a random cell arrangement ( Fig. 6d,e ), the adjacent cells mean the cells that are located within a radius of 0.5. In the multiple cell model with a hexagonal cell arrangement ( Supplementary Fig. 14c ), the adjacent cells mean the six immediate neighbours. The sum of the expression levels in adjacent cells was divided by 6, so that it would be easier to compare the random cell arrangement ( Fig. 6d,e ) with the hexagonal cell arrangement ( Supplementary Fig. 14c ). As for the model for the aTR cells and aTRLF cells that were treated with Dox ( Fig. 7b ), the following equations were used instead of equations (2, 6, 9 and 14). Bifurcation diagrams of the models with two cells were produced by XPPAUT. Numerical simulations of the models were performed by using Matlab's ode45 solver until the system reaches a steady state. How to cite this article: Matsuda, M. et al. Synthetic lateral inhibition governs cell-type bifurcation with robust ratios. Nat. Commun. 6:6195 doi: 10.1038/ncomms7195 (2015).